A non-conserved miRNA regulates lysosomal function and impacts on a human lysosomal storage disorder Sulfatases are key enzymatic regulators of sulfate homeostasis with several biological functions including degradation of glycosaminoglycans (GAGs) and other macromolecules in lysosomes. In a severe lysosomal storage disorder, multiple sulfatase deficiency (MSD), global sulfatase activity is deficient due to mutations in the sulfatase-modifying factor 1 ( SUMF1 ) gene, encoding the essential activator of all sulfatases. We identify a novel regulatory layer of sulfate metabolism mediated by a microRNA. miR-95 depletes SUMF1 protein levels and suppresses sulfatase activity, causing the disruption of proteoglycan catabolism and lysosomal function. This blocks autophagy-mediated degradation, causing cytoplasmic accumulation of autophagosomes and autophagic substrates. By targeting miR-95 in cells from MSD patients, we can effectively increase residual SUMF1 expression, allowing for reactivation of sulfatase activity and increased clearance of sulfated GAGs. The identification of this regulatory mechanism opens the opportunity for a unique therapeutic approach in MSD patients where the need for exogenous enzyme replacement is circumvented. Maintaining the required biological ratio of sulfated versus non-sulfated molecules in the cell is critical for several biological processes ranging from fetal development and hormone metabolism to growth factor signalling, bone remodelling and degradation of macromolecules [1] , [2] , [3] , [4] , [5] . Thus, sulfate homeostasis is highly dynamic and tightly regulated by multiple enzymes including a large family of sulfatase enzymes that hydrolyse sulfate esters from many substrates, including sulfolipids, steroid sulfates and glycosaminoglycans (GAGs) [6] . To date, 17 human sulfatases are known, broadly categorized into two main groups, exerting their enzymatic activity either at a neutral or an acidic pH. The latter category comprises the lysosomal sulfatases, primarily involved in the catabolism of sulfated protein substrates within lysosomes [7] . Importantly, inadequate lysosomal sulfatase activity causes substrate accumulation, ultimately leading to lysosomal dysfunction, which impacts on several cellular pathways. Macroautophagy (hereafter referred to as autophagy) is a lysosome-dependent cellular degradation process in which proteins and organelles are degraded through their integration into autophagosomes followed by autophagosome–lysosome fusion. Autophagy is vital for basal homeostasis and for promoting survival during cellular stress by nutrient recycling and removal of damaged proteins and organelles [8] . Importantly, lysosomal dysfunction is tightly linked to defective protein clearance via the autophagy pathway [9] , [10] , [11] . The importance of lysosomal sulfatases in human metabolism is underscored by the discovery of several inherited diseases caused by impaired desulfation, including a subgroup of lysosomal storage disorders (LSDs) called the mucopolysaccharidoses. These LSDs are characterized by defective catabolism of lysosomal GAGs, and clinical symptoms relate mainly to GAG deposition in multiple tissues [7] , [10] . In a particularly severe LSD, multiple sulfatase deficiency (MSD), all sulfatase activities are simultaneously defective due to mutations in the sulfatase-modifying factor 1 ( SUMF1 ) gene. SUMF1 encodes a C α -formylglycine (FGly)-generating enzyme (also known as FGE) responsible for a key post-translational modification of a highly conserved cysteine residue within the active site of all sulfatases, essential for their activation [12] , [13] , [14] . The clinical picture of MSD is complex and combines the symptoms of individual sulfatase deficiencies including severe neurodegeneration, skeletal abnormalities, facial dysmorphism, organomegaly and premature death [7] . Recent studies, including the generation of the Sumf1 −/− mouse, have elucidated important links between the pathogenesis of MSD and inhibition of the autophagy pathway [4] , [9] . MicroRNAs (miRNAs) comprise one class of a growing number of endogenous non-coding RNA subtypes, which were discovered a little more than a decade ago [15] . These single-stranded RNAs are post-transcriptional gene regulators, which have received much attention due to their critical regulatory impact on biological functions related to development, proliferation, stress signalling and metabolism [15] , [16] . Although many miRNAs have modest effects on gene expression, several studies have elucidated major regulatory functions for miRNAs, including the miR-17-92/miR-106b-25 clusters in embryonic development [17] and miR-133 in cardiac and skeletal muscle development [18] , [19] . Not surprisingly, miRNAs have been causally linked to diseases ranging from neurological disorders and infectious diseases to metabolic disorders and cancers [20] . The ability of single miRNAs to simultaneously regulate multiple targets within a specific biological network or pathway presents a potential advantage for miRNA-targeting strategies in the therapy of human disease. In this study, we uncover a novel mechanism by which a miRNA can regulate sulfate homeostasis and lysosomal function. miR-95, by targeting the key activator of all cellular sulfatases, SUMF1 , can effectively shut down sulfatase activity and disrupt lysosomal function. This causes a severe block in autophagy-mediated degradation, demonstrated by the build-up of autophagosomes, autophagic markers and autophagic substrates. Intriguingly, we show that by targeting miR-95 in cells isolated from MSD patients, which harbour hypomorphic mutations in the SUMF1 gene, we can effectively increase SUMF1 proteins levels and residual SUMF1 activity. This leads to an enhanced clearance of total cellular sulfated GAGs, indicating a potential therapeutic advantage for miR-95 targeting in the treatment of MSD. miR-95 inhibits late-stage autophagy In a previously described functional screen, we identified several miRNAs, which can regulate the autophagy pathway in human MCF-7 cells [21] . A top candidate repressor of autophagy, miR-95, has previously been investigated in few studies only [22] , [23] , [24] , [25] . We found that miR-95 is differentially expressed across human tissues with the highest expression in skeletal muscle and brain. miR-95 is an intronic miRNA and its host gene, actin binding LIM protein 2 ( ABLIM2 ), displays a similar expression profile ( Supplementary Fig. 1a ). Interestingly, the sequence encoding miR-95 overlaps a LINE-2 (long interspersed nuclear element 2) and its conservation is limited to the primate lineage and a few other higher mammals, suggesting its relatively recent evolutionary emergence ( Supplementary Fig. 1b ). We found that the overexpression of miR-95 in MCF-7 cells effectively increased protein levels of LC3II, a hallmark of autophagy ( Fig. 1a ). Likewise, miR-95 caused accumulation of green fluorescent protein (GFP)-LC3 puncta, a marker of autophagosomes ( Fig. 1c and Supplementary Fig. 2a ). Since autophagosome accumulation can result either from increased de novo autophagosome biosynthesis or inhibition of autophagic flux, we distinguished between these possibilities by use of the lysosomal inhibitor, Bafilomycin A1. Importantly, miR-95 did not further increase the LC3II levels and GFP-LC3 puncta during Bafilomycin A1 treatment, indicating a miR-95-induced degradation block at a late step in the autophagy pathway ( Fig. 1b,d and Supplementary Fig. 2a ). To further assess the effect of miR-95, we quantified the levels of p62, a protein incorporated into autophagosomes and degraded in autolysosomes [26] . The increase in p62 mediated by miR-95 further confirmed a block in autophagic flux ( Fig. 1a,b ). Using a previously described luciferase-based autophagic flux assay, based on a fusion between LC3 and renilla luciferase (RLuc), we monitored the degradation of RLuc-LC3 wt relative to a mutated RLuc-LC3 G120A , which does not undergo autophagosomal localization [27] . At three different time points after transfection, miR-95 significantly increased the RLuc-LC3 wt /RLuc-LC3 G120A ratio, indicating the inhibition of autophagic flux ( Fig. 1e ). Assessing this defect at the ultrastructural level by transmission electron microscopy (TEM), we observed that miR-95 induced the accumulation of both initial (AVi) and degradative (AVd) autophagic vacuoles in MCF-7 cells ( Fig. 1g and Supplementary Fig. 2b ). As a block in the autophagy-mediated degradation often is accompanied by an accumulation of autophagy substrates, we assessed the total cellular levels of ubiquitin and mitochondria, both of which were increased upon miR-95 overexpression ( Fig. 1f,h ). Taken together, these data suggest that miR-95 effectively blocks autophagy at a relatively late step in the pathway, after the formation and maturation of the autophagosome. This is accompanied by a build-up of both early and late autophagosomes, autophagic markers and autophagy substrates. After 4 days of transfection, miR-95 inhibited the cellular growth rate ( Fig. 1i and Supplementary Fig. 2c ). At this time point, no significant effect was seen on the level of apoptosis, as assessed by cleavage of the caspase substrate PARP ( Supplementary Fig. 2d ). Furthermore, analysis of cell cycle distribution by incorporation of the modified nucleoside, EdU, revealed that miR-95 effectively reduced the proportion of cells in S-phase ( Fig. 1j ). 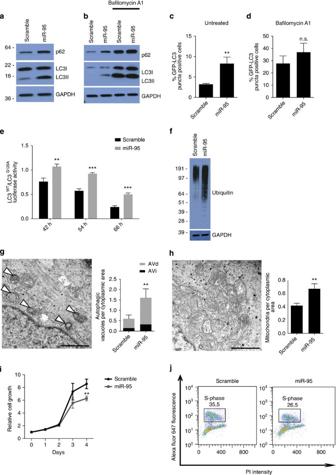Figure 1: miR-95 inhibits autophagic flux and represses cellular growth. (a,b) Western blot in MCF-7 cells of LC3 and p62 proteins 72 h after transfection in the absence or presence of Bafilomycin A1 (three independent experiments) (c,d) Quantification of eGFP-LC3 puncta in MCF-7 cells stably expressing eGFP-LC3 72 h after transfection in the absence or presence of Bafilomycin A1 (n=4–5 wells, three independent experiments). Data are mean+s.d. from one representative experiment. (e) MCF-7 cells stably expressing RLuc-LC3WTor RLuc-LC3G120Awere transfected and luciferase activity ratios were assessed at indicated time points after transfection (n=4 wells, three independent experiments). Data are mean+s.d. from one representative experiment. (f) Western blot of total ubiquitin in MCF-7 cells 72 h after transfection (three independent experiments). (g) Left: representative image showing autophagic vacuoles (indicated by arrowheads) in miR-95-transfected cells. Scale bar, 1 μm. Right: quantification of AVi and AVd per cytoplasmic area from MCF-7 cells 72 h after transfection (n=30–35 cells per sample). Data are mean+s.e.m. (h) Left: representative image from miR-95-transfected cells showing mitochondria. Scale bar, 1 μm. Right: quantification of mitochondria per cytoplasmic area in MCF-7 cells 72 h after transfection (n=30–35 cells per sample). Data are mean+s.e.m. (i) Quantification of cellular growth by crystal violet analysis on four consecutive days after transfection in MCF-7 cells (n=4 wells, two independent experiments). Data are mean+s.d. from one representative experiment. (j) Quantification of cell cycle distribution in MCF-7 cells 4 days after transfection by the Click-IT Plus EdU Alexa Fluor flow cytometry assay kit (two independent experiments). n.s., non-significant. Figure 1: miR-95 inhibits autophagic flux and represses cellular growth. ( a , b ) Western blot in MCF-7 cells of LC3 and p62 proteins 72 h after transfection in the absence or presence of Bafilomycin A1 (three independent experiments) ( c , d ) Quantification of eGFP-LC3 puncta in MCF-7 cells stably expressing eGFP-LC3 72 h after transfection in the absence or presence of Bafilomycin A1 ( n =4–5 wells, three independent experiments). Data are mean+s.d. from one representative experiment. ( e ) MCF-7 cells stably expressing RLuc-LC3 WT or RLuc-LC3 G120A were transfected and luciferase activity ratios were assessed at indicated time points after transfection ( n =4 wells, three independent experiments). Data are mean+s.d. from one representative experiment. ( f ) Western blot of total ubiquitin in MCF-7 cells 72 h after transfection (three independent experiments). ( g ) Left: representative image showing autophagic vacuoles (indicated by arrowheads) in miR-95-transfected cells. Scale bar, 1 μm. Right: quantification of AVi and AVd per cytoplasmic area from MCF-7 cells 72 h after transfection ( n =30–35 cells per sample). Data are mean+s.e.m. ( h ) Left: representative image from miR-95-transfected cells showing mitochondria. Scale bar, 1 μm. Right: quantification of mitochondria per cytoplasmic area in MCF-7 cells 72 h after transfection ( n =30–35 cells per sample). Data are mean+s.e.m. ( i ) Quantification of cellular growth by crystal violet analysis on four consecutive days after transfection in MCF-7 cells ( n =4 wells, two independent experiments). Data are mean+s.d. from one representative experiment. ( j ) Quantification of cell cycle distribution in MCF-7 cells 4 days after transfection by the Click-IT Plus EdU Alexa Fluor flow cytometry assay kit (two independent experiments). n.s., non-significant. Full size image Transcriptome profiling identifies SUMF1 as a miR-95 target To clarify the underlying mechanism for the miR-95-induced block in autophagy-mediated degradation, we performed transcriptome profiling 24 h after the overexpression of miR-95 or a scramble control in MCF-7 cells. We have previously used this approach for the successful identification of multiple miRNA targets [21] , [28] , [29] . Out of 1,336 differentially expressed genes, 1,087 were downregulated, while 249 were upregulated (false discovery rate, FDR≤0,1; Supplementary Table 1 ). We found a significant enrichment of potential miR-95-binding sites (seed sites) within the 3′UTRs of the downregulated transcripts relative to the upregulated transcripts or transcripts with no change in expression level ( Fig. 2a ), indicating a high likelihood for identification of direct miR-95 targets by this approach. 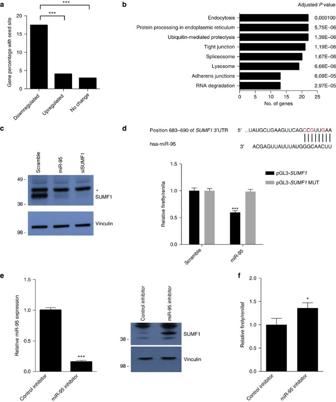Figure 2: Transcriptome profiling identifies SUMF1 as a direct miR-95 target. (a) Seed site enrichment analysis. The proportion of transcripts in the up, down and no change sets containing miR-95 seed sites (see Methods). (b) KEGG analysis of enriched pathways among deregulated genes after miR-95 overexpression relative to scramble control (see Methods). (c) Western blot of SUMF1 protein 72 h after transfection in MCF-7 cells (three independent experiments) * indicates an unspecific band. (d) Upper panel: predicted binding between miR-95 andSUMF13′UTR. Bases shown in red were mutated in the pGL3-SUMF1 MUT construct. Lower panel: luciferase reporter assay 24 h after transfection with pGL3-SUMF1 or pGL3-SUMF1 MUT and pRLTK control plasmid, co-transfected with either miR-95 or scramble control in HEK cells (n=4 wells, three independent experiments). Data are mean+s.d. from one representative experiment. (e) Left: qRT–PCR assessment of miR-95 expression in HEK cells stably transduced with control or miR-95 inhibitor plasmids. Data are plotted relative to housekeeping and are mean+s.d. (n=3, two independent experiments). Right: western blot of SUMF1 protein in stably transduced HEK cells. (f) Transient co-transfection of control or miR-95 inhibitor plasmid, pGL3-SUMF1 and pRLTK followed by luciferase reporter assay 48 h after transfection (n=4 wells, three independent experiments). Data are mean+s.d. from one representative experiment. Figure 2: Transcriptome profiling identifies SUMF1 as a direct miR-95 target. ( a ) Seed site enrichment analysis. The proportion of transcripts in the up, down and no change sets containing miR-95 seed sites (see Methods). ( b ) KEGG analysis of enriched pathways among deregulated genes after miR-95 overexpression relative to scramble control (see Methods). ( c ) Western blot of SUMF1 protein 72 h after transfection in MCF-7 cells (three independent experiments) * indicates an unspecific band. ( d ) Upper panel: predicted binding between miR-95 and SUMF1 3′UTR. Bases shown in red were mutated in the pGL3-SUMF1 MUT construct. Lower panel: luciferase reporter assay 24 h after transfection with pGL3-SUMF1 or pGL3-SUMF1 MUT and pRLTK control plasmid, co-transfected with either miR-95 or scramble control in HEK cells ( n =4 wells, three independent experiments). Data are mean+s.d. from one representative experiment. ( e ) Left: qRT–PCR assessment of miR-95 expression in HEK cells stably transduced with control or miR-95 inhibitor plasmids. Data are plotted relative to housekeeping and are mean+s.d. ( n =3, two independent experiments). Right: western blot of SUMF1 protein in stably transduced HEK cells. ( f ) Transient co-transfection of control or miR-95 inhibitor plasmid, pGL3-SUMF1 and pRLTK followed by luciferase reporter assay 48 h after transfection ( n =4 wells, three independent experiments). Data are mean+s.d. from one representative experiment. Full size image Using the KEGG pathway database, we identified functional gene categories, enriched among all deregulated genes after the overexpression of miR-95. Interestingly, while there was no enrichment of autophagy-related genes, we observed a highly significant enrichment for closely related pathways such as endocytosis and lysosomal function ( Fig. 2b ). We validated the microarray data by quantitative reverse transcriptase-PCR (qRT–PCR) for 10 transcripts, selected based on interesting biological functions related to lysosomal function, autophagy, proliferation, apoptosis, cell cycle regulation and mitochondrial function. This included the previously published miR-95 target, Snx-1 ( Supplementary Fig. 3a ). Three of these genes, ATG2B , PSEN1 and SUMF1 were selected for further validation at the protein level based on previously described links to autophagy and/or lysosomal function. While modest effects were observed on ATG2B and PSEN1 protein levels ( Supplementary Fig. 3b ), a very striking downregulation of SUMF1 protein levels was observedupon miR-95 overexpression ( Fig. 2c ). Since miRNAs rarely achieve such profound deregulation of their targets, we were intrigued to pursue this further. The SUMF1 3′UTR contains an 8mer seed match at position 683–690, which is predicted to bind miR-95 ( www.targetscan.org ; Fig. 2d ). To address whether miR-95 directly regulates SUMF1 via binding to this site, we cloned a luciferase reporter vector containing a 450-bp fragment of the SUMF1 3′UTR. We used HEK cells for all plasmid transfections due to higher transfection efficiency in this cell line. While miR-95 significantly repressed luciferase activity from this construct, this repression was fully abolished upon mutation of three bases within the miR-95 seed match ( Fig. 2d ). Importantly, the inhibition of endogenous miR-95 resulted in a clear increase in SUMF1 protein levels ( Fig. 2e ) and a significant derepression of luciferase activity from the SUMF1 3′UTR reporter construct ( Fig. 2f ). Together these findings confirm that SUMF1 is a direct endogenous target of miR-95. miR-95 impacts on sulfatase activity and lysosomal function Sulfation represents an important protein modification, with diverse roles in several biological settings [1] , [2] , [3] . Importantly, sulfate metabolism is highly dynamic and sulfate groups are efficiently removed from sulfated proteins by a large family of sulfatase enzymes [7] . All sulfatases require activation by SUMF1, which post-translationally modifies a conserved cysteine residue in the active pocket to FGly ( Fig. 3a ). Thus, we hypothesized that miR-95, through its regulation of SUMF1 , could regulate sulfatase activity. To functionally assess this, we measured the enzymatic activity of the lysosomal sulfatase Arylsulfatase B (ARSB). Indeed, co-expressing miR-95 together with an ARSB-expressing plasmid confirmed that miR-95 could efficiently repress ARSB activity to an extent comparable to that of short interfering RNA (siRNA)-mediated depletion of SUMF1 ( Figs 2c , 3b ). In addition, the low level of endogenous ARSB activity was significantly increased by miR-95 inhibition ( Fig. 3c ). These findings were confirmed with respect to two additional sulfatases, the lysosomal ARSA and the non-lysosomal ARSC ( Supplementary Fig. 4a,b ). To investigate whether miR-95 affected protein levels of sulfatases, we performed western blotting for ARSB. While the ARSB precursor was not affected, the mature ARSB protein was profoundly decreased by both miR-95 and siSUMF1 ( Supplementary Fig. 4c,d ). This can likely be ascribed to the reduced stability of ARSB in the absence of the formylglycine modification, as observed previously in MSD [30] . miR-95, similar to siSUMF1, did not affect ARSA, ARSB and ARSC mRNAs levels, excluding the possibility of direct regulation of the sulfatase transcripts by miR-95 ( Supplementary Fig. 4e ). 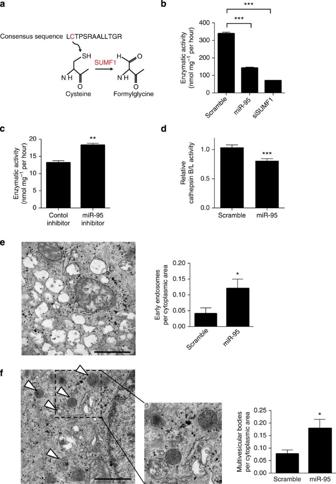Figure 3: miR-95 regulates sulfatase activity and lysosomal function. (a) Schematic showing the SUMF1-mediated post-translational modification of a conserved cysteine to a formylglycine located in a consensus sequence of the sulfatase active pocket. (b) HEK cells were co-transfected with indicated siRNA or miRNA and pcDNA3-ARSB and assessed for ARSB enzymatic activity 72 h post transfection (n=3, two independent experiments). Data are mean+s.d. from one representative experiment. (c) HEK cells stably transduced with control or miR-95-knockdown vectors were assessed for ARSB enzymatic activity 1 week after viral transduction (n=3, two independent experiments). Data are mean+s.d. from one representative experiment. (d) Cathepsin B/L activity was measured 72 h after transfection and normalized to total protein levels (n=4–5 wells, four independent experiments). Data are mean+s.e.m. from four pooled experiments. (e) Left: representative TEM image showing early endosomes in miR-95-transfected cells. Scale bar, 1 μm. Right: quantification of early endosomes per cytoplasmic area from MCF-7 cells 72 h after transfection (n=30–35 cells/sample). Data are mean+s.e.m. (f) Left: representative TEM image showing multivesicular bodies (denoted by arrowheads) in miR-95-transfected cells. Scale bar=1 μm. Right: quantification of multivesicular bodies per cytoplasmic area from MCF-7 cells 72 h after transfection (n=30–35 cells per sample). Data are mean+s.e.m. Figure 3: miR-95 regulates sulfatase activity and lysosomal function. ( a ) Schematic showing the SUMF1-mediated post-translational modification of a conserved cysteine to a formylglycine located in a consensus sequence of the sulfatase active pocket. ( b ) HEK cells were co-transfected with indicated siRNA or miRNA and pcDNA3-ARSB and assessed for ARSB enzymatic activity 72 h post transfection ( n =3, two independent experiments). Data are mean+s.d. from one representative experiment. ( c ) HEK cells stably transduced with control or miR-95-knockdown vectors were assessed for ARSB enzymatic activity 1 week after viral transduction ( n =3, two independent experiments). Data are mean+s.d. from one representative experiment. ( d ) Cathepsin B/L activity was measured 72 h after transfection and normalized to total protein levels ( n =4–5 wells, four independent experiments). Data are mean+s.e.m. from four pooled experiments. ( e ) Left: representative TEM image showing early endosomes in miR-95-transfected cells. Scale bar, 1 μm. Right: quantification of early endosomes per cytoplasmic area from MCF-7 cells 72 h after transfection ( n =30–35 cells/sample). Data are mean+s.e.m. ( f ) Left: representative TEM image showing multivesicular bodies (denoted by arrowheads) in miR-95-transfected cells. Scale bar=1 μm. Right: quantification of multivesicular bodies per cytoplasmic area from MCF-7 cells 72 h after transfection ( n =30–35 cells per sample). Data are mean+s.e.m. Full size image Lysosomal desulfation of proteoglycans and other highly sulfated substrates is a prerequisite for their further degradation in the lysosomes [31] . A block in the lysosomal sulfatase activity, causing lysosomal accumulation of sulfated substrates will ultimately disrupt lysosomal function, which can be reflected by an impact on the enzymatic function of other lysosomal enzymes. To investigate this, we measured the activity of the lysosomal proteases cathepsin B and L. Indeed, miR-95 significantly decreased cathepsin activity by 20% after 72 h transfection, indicating that miR-95 not only disrupts lysosomal sulfatases, but also affects general lysosomal function ( Fig. 3d ). Remarkably, several additional genes identified by our transcriptomic profiling were related to lysosomal function ( Fig. 2b and Supplementary Table 1 ), indicating additional either primary or secondary targets of miR-95 that could impact on lysosomal function. Interestingly, as indicated by our TEM analysis, transfection of miR-95 significantly increased the level of early and late endosomes/multivesicular bodies relative to the scramble control, suggesting a possible block in the endocytosis pathway ( Fig. 3e,f ). Since both endosomal and autophagic pathways converge at the level of the lysosome, these data further support the hypothesis that the main mechanism for miR-95 occurs at the level of lysosomal function. Depletion of SUMF1 phenocopies effects of miR-95 To assess the biological importance of SUMF1 as a miR-95 target, we performed siRNA-mediated knockdown of SUMF1 and assessed the effects on all autophagy-related phenotypes in MCF-7 cells. Indeed, the depletion of SUMF1 effectively inhibited the autophagic flux as measured by the RLuc-based assay ( Fig. 4a ). Furthermore, siSUMF1 significantly increased the GFP-LC3 puncta ( Fig. 4b ) and caused the accumulation of p62 and LC3II protein levels ( Fig. 4c ). siSUMF1, like miR-95, caused a build-up of AVi and AVd as assessed by TEM ( Fig. 4e ) and moreover, autophagic substrates such as mitochondria and total ubiquitin levels were increased by the knockdown of SUMF1 ( Fig. 4d,f ). Notably, the degree of these phenotypic observations was highly comparable to the effects of miR-95 and the knockdown efficiency of the siRNA and miRNA were highly similar ( Fig. 2c ), indicating that SUMF1 is likely a main target of miR-95. 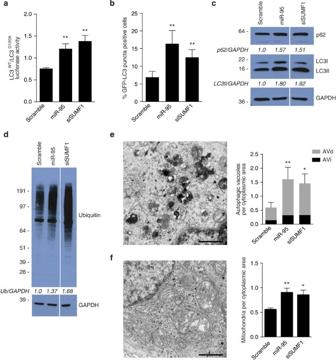Figure 4: siRNA-mediated depletion of SUMF1 phenocopies miR-95 overexpression. (a) MCF-7 cells stably expressing RLuc-LC3WTor RLuc-LC3G120Awere transfected and luciferase activity ratios were assessed at 42 h after transfection (n=4 wells, three independent experiments). Data are mean+s.d. from a representative experiment. (b) Quantification of eGFP-LC3 puncta in MCF-7 cells stably expressing eGFP-LC3 72 h after transfection (n=4-5 wells, three independent experiments). Data are mean+s.d. from one representative experiment. (c) Western blot in MCF-7 cells of LC3 and p62 proteins 72 h after transfection (three independent experiments). Quantifications relative to GAPDH are shown below the bands. (d) Western blot of total ubiquitin in MCF-7 cells 72 h after transfection. Quantifications relative to GAPDH are shown. (e) Left: representative image from the miR-95-transfected cells showing autophagic vacuoles. Scale bar, 1 μm. Right: quantification of AVi and AVd per cytoplasmic area in MCF-7 cells 72 h after transfection (n=30–35 cells per sample). Data are mean+s.e.m. (f) Left: representative image from miR-95-transfected cells showing mitochondria. Scale bar, 1 μm. Right: quantification of mitochondria per cytoplasmic area in MCF-7 cells 72 h after transfection (n=30–35 cells per sample). Data are mean+s.e.m. Figure 4: siRNA-mediated depletion of SUMF1 phenocopies miR-95 overexpression. ( a ) MCF-7 cells stably expressing RLuc-LC3 WT or RLuc-LC3 G120A were transfected and luciferase activity ratios were assessed at 42 h after transfection ( n =4 wells, three independent experiments). Data are mean+s.d. from a representative experiment. ( b ) Quantification of eGFP-LC3 puncta in MCF-7 cells stably expressing eGFP-LC3 72 h after transfection ( n =4-5 wells, three independent experiments). Data are mean+s.d. from one representative experiment. ( c ) Western blot in MCF-7 cells of LC3 and p62 proteins 72 h after transfection (three independent experiments). Quantifications relative to GAPDH are shown below the bands. ( d ) Western blot of total ubiquitin in MCF-7 cells 72 h after transfection. Quantifications relative to GAPDH are shown. ( e ) Left: representative image from the miR-95-transfected cells showing autophagic vacuoles. Scale bar, 1 μm. Right: quantification of AVi and AVd per cytoplasmic area in MCF-7 cells 72 h after transfection ( n =30–35 cells per sample). Data are mean+s.e.m. ( f ) Left: representative image from miR-95-transfected cells showing mitochondria. Scale bar, 1 μm. Right: quantification of mitochondria per cytoplasmic area in MCF-7 cells 72 h after transfection ( n =30–35 cells per sample). Data are mean+s.e.m. Full size image miR-95 inhibition in MSD cells restores sulfatase function The importance of lysosomal sulfatases in human metabolism is underlined by the study of inherited diseases resulting from defects in sulfatase function [31] . Since SUMF1 is an essential activator of all cellular sulfatases, mutations in this gene cause the most severe disease variant, MSD, in which all sulfatase activity is severely reduced [12] , [32] . To assess the physiological importance of miR-95 in relation to MSD, we stably knocked down endogenous miR-95 in two lymphoblast and four fibroblast lines derived from six MSD patients harbouring different mutations in the SUMF1 gene (see Methods). Since MSD mutations are hypomorphic, sulfatase activity is suppressed to varying extents but not fully abolished, and thus we reasoned that the inhibition of miR-95 could be utilized as a tool to increase residual SUMF1 function. Indeed, stable miR-95 inhibition could effectively increase SUMF1 expression levels in fibroblasts and lymphoblasts from all six MSD patients ( Fig. 5a ). To address whether this enhanced SUMF1 expression was functional, we measured the ARSB activity in three MSD fibroblast lines, BA 956, BA 919 and 0322001. In all three lines, stable miR-95 inhibition caused a consistent increase in ARSB activity ( Fig. 5b ). The downregulation of miR-95 levels was confirmed in each of the three cell types by qRT–PCR ( Supplementary Fig. 5 ). 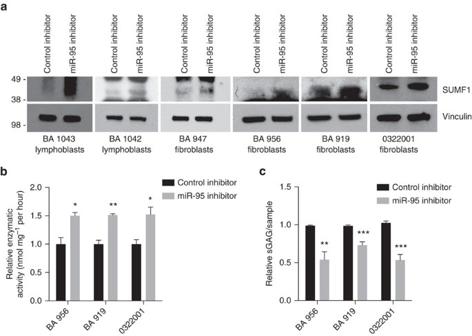Figure 5: Inhibition of miR-95 in MSD cells can raise residual SUMF1 expression and activity. (a) Two MSD lymphoblast lines (BA 1042 and BA 1043) and four MSD fibroblast lines (BA 947, BA 956, BA 919 and 0322001) were stably transduced with control or miR-95 inhibitor and assessed for SUMF1 expression by western blotting within 1 week after transduction. (b) Assessment of ARSB enzymatic activity in three MSD fibroblast lines stably transduced with control or miR-95 inhibitor (n=3, two independent experiments). Data are mean+s.d. from one representative experiment. (c) Assessment of total cellular sulfated GAG concentration in three stable MSD control or miR-95-knockdown cells (n=3 wells, four independent experiments). Data are mean+s.e.m. from four pooled experiments. Figure 5: Inhibition of miR-95 in MSD cells can raise residual SUMF1 expression and activity. ( a ) Two MSD lymphoblast lines (BA 1042 and BA 1043) and four MSD fibroblast lines (BA 947, BA 956, BA 919 and 0322001) were stably transduced with control or miR-95 inhibitor and assessed for SUMF1 expression by western blotting within 1 week after transduction. ( b ) Assessment of ARSB enzymatic activity in three MSD fibroblast lines stably transduced with control or miR-95 inhibitor ( n =3, two independent experiments). Data are mean+s.d. from one representative experiment. ( c ) Assessment of total cellular sulfated GAG concentration in three stable MSD control or miR-95-knockdown cells ( n =3 wells, four independent experiments). Data are mean+s.e.m. from four pooled experiments. Full size image Free and proteoglycan-bound GAG chains are highly modified by sulfation and are the main substrates for lysosomal sulfatases. Hence, GAGs are the primary substrate type seen to accumulate in multiple tissues from the Sumf1 −/− MSD mouse model as well in MSD patients [4] , [33] . To test whether SUMF1 and thereby sulfatase reactivation by miR-95 inhibition could affect cellular levels of sulfated GAGs, we extracted and quantified total sulfated GAGs from MSD fibroblasts. Importantly, the inhibition of miR-95 in all three MSD fibroblast lines decreased the levels of total sulfated GAGs ( Fig. 5c ). Altogether, these data indicate that inhibition of miR-95 can be used as a tool in MSD to enhance SUMF1 expression and partially rescue sulfatase activity, leading to a reduced level of total cellular sulfated GAGs. In this study, we have identified a non-conserved miRNA, which can convey a unique molecular switch in sulfate metabolism by shutting down an entire family of cellular sulfatases at once through the regulation of a single target. Remarkably, the non-redundant function of SUMF1 is clearly illustrated by the complete lack of any detectable sulfatase activity in the Sumf1 −/− mouse [4] , rendering this system highly vulnerable to manipulation by regulating factors such as miRNAs. Indeed, the robust depletion of SUMF1 protein by miR-95 causes the effective suppression of downstream lysosomal sulfatase activity, affecting not only proteoglycan catabolism, but also general lysosomal function. Importantly, miR-95 causes a block in autophagy-mediated degradation, resulting in the cytoplasmic build-up of autophagosomes and autophagic substrates. The similarities between our findings and the phenotypes seen in the brain and in cultured MEFs from the Sumf1 −/− mouse are striking. This MSD mouse model displays accumulation of autophagosomes and autophagic substrates including mitochondria, polyubiquitinated proteins and p62, as a result of defective autophagosome–lysosome fusion [9] . Excess lysosomal storage of GAGs in several organs of the Sumf1 −/− mouse is likely causative of most disease-related phenotypes, leading to frequent early mortality [4] . The antiproliferative role of miR-95 that we observed in MCF-7 cells could be a result of general loss of sulfatase function or perhaps more specifically due to lysosomal damage and autophagic block; however, this will require further mechanistic investigation. Interestingly, the role of miR-95 with respect to cellular proliferation and cancer seems to be highly tissue dependent. While it was suggested to have proproliferative function in prostate, lung and pancreatic cancers [22] , [24] , [34] , its downregulation in head and neck cancers as well as in glioblastomas suggests a tumour-suppressive role for miR-95 in these tissues [35] , [36] . The absence of miR-95 in mice, flies and worms indicates the relatively late evolutionary emergence of this miRNA. Indeed, its species conservation is limited to primates and some other higher mammals. Moreover, its derivation from a LINE-2 element could indicate that retrotransposition has been a driving force in the late emergence of miR-95 (ref. 37 ). In contrast, SUMF1 is highly conserved from prokaryotes to eukaryotes [7] . However, the miR-95-binding site in its 3′UTR has emerged in the primate lineage, perhaps indicating that increasing demands for a more tightly controlled sulfate metabolism in higher organisms have favoured the evolution of this unique layer of regulation. Indeed, the need for increased complexity of sulfatase regulation during evolution is further supported by the large expansion in sulfatase family members from bacteria and lower eukaryotes to higher eukaryotes [7] . Although we observed a trend towards a negative correlation between miR-95 and SUMF1 expression in human tissues ( Supplementary Fig. 1a ), this correlation was not statistically significant, indicating the presence of additional regulators of SUMF1 expression. LSDs comprise a large and diverse group of rare genetic metabolic disorders resulting from defects in lysosomal function [38] . The combined incidence of LSDs is 1:5,000 live births; however, the precise figure is likely larger when undiagnosed and misdiagnosed cases are considered. A role for miRNAs in LSDs is largely unexplored and although one study has profiled miRNAs in fibroblasts from Niemann–Pick patients [39] , the concept of a miRNA functionally impacting on LSDs is, to our knowledge, not previously known. Intriguingly, in this study, we shed light on the possibility for targeting miR-95 therapeutically in the setting of MSD, where hypomorphic mutations in the SUMF1 gene severely reduce sulfatase activity [12] , [13] . Several independent SUMF1 mutations have been identified, which span the length of the gene and while only few are found to affect catalytic activity and/or substrate binding, the vast majority of identified mutations cause a reduction in SUMF1 protein stability [40] , [41] . By inhibiting miR-95 in cells isolated from MSD patients, we can effectively raise residual SUMF1 protein levels, partially restoring downstream sulfatase activity and increasing cellular clearance of sulfated GAG substrates. While the past and current developments of therapeutic approaches have focused on methods for the reintroduction of SUMF1 and/or sulfatase enzymes [40] , we present here the possibility for a novel therapeutic strategy where the need for exogenous enzyme replacement is circumvented. The ability to inhibit miRNA activity using antisense oligonucleotides provides novel opportunities for intervening in disease processes. Since current therapy options for LSDs including enzyme replacement and haematopoietic stem cell therapies have had only modest success, novel therapeutic approaches are in high demand [42] . Anti-miRs with a variety of modifications have been developed to increase potency, specificity and bioavailability, including the locked nucleic acid modification, which can be delivered systemically with little or no toxicity [43] , [44] . The success of the locked nucleic acid-based miR-122 antimiR in phase II clinical trials for hepatitis C virus treatment illustrates a promising potential for antimiR-based therapeutics [45] . Analysis of the SUMF1 mutations in MSD revealed multiple types including missense, nonsense, deletions and splice mutations [32] . The effect of these mutations on enzyme activity is variable as is the clinical picture in MSD patients; however, a lack of genotype–phenotype correlation indicates the existence of additional causative factors, either genetic or non-genetic, which could contribute to disease pathogenesis [32] . This leads to the speculation that miR-95, via its regulation of SUMF1, and perhaps also additional targets related to lysosomal function, could contribute to the pathogenesis MSD or other LSDs. Since this feature of impaired autophagy and escalation of cytoplasmic protein aggregation is shared between LSDs and the more common neurodegenerative diseases, including Alzheimers, Parkinsons and Huntingtons disorders, the targeting of miR-95 and other as yet unidentified miRNAs with functional implications in this pathway present a promising area for future therapeutic research. Cell culture MCF-7 eGFP-LC3 (ref. 46 ) MCF-7 RLuc-LC3 WT and MCF-7 RLuc-LC3 G120A (ref. 27 ) cells were propagated in RPMI 1640 (Invitrogen) supplemented with 6% fetal bovine serum (FBS), 100 U ml −1 penicillin and 100 μg ml −1 streptomycin (P/S). HEK 293 cells (used for plasmid transfections due to higher transfection efficiency than MCF-7) were propagated in DMEM supplemented with 10% FBS and P/S and were purchased from ATCC. MSD fibroblasts and lymphoblasts BA 947, BA 956, BA 919, BA 1042 and BA 1043 are previously described [32] , [47] . Fibroblasts (0322001) are not previously described and contain the SUMF1 gene mutations: c.1033C>T+c.653G>A giving rise to the predicted amino-acid changes: p.R345C+p.C218Y. BA 956, BA 919 and 0322001 (FFFO322001) were kindly provided by the Telethon Network of Genetic Biobanks. BA 947 were propagated in alpha-MEM supplemented with 20% FBS and P/S, BA 1042 and BA 1043 were propagated in RPMI 1640 supplemented with 20% FBS and P/S. BA 956, BA 919 and 0322001 were propagated in RPMI 1640 supplemented with 10% FBS and P/S. Cell growth MCF-7 cells were seeded in 24-well plates and transfected the following day with 50 nM miR-95 or Scramble control. Cells were fixed at indicated time points in 4% paraformaldehyde, stained in a 0.1% crystal violet solution and resuspended in 10% acetic acid. Sample absorbance was measured at 620 nm. EdU detection Cells were incubated in 33 μM EdU for 25 min and analysed with the Click-IT Plus EdU flow cytometry assay according to the manufacturer’s protocol (Molecular Probes). Cells were counterstained with propidium iodide for DNA content and the EdU Alexa Fluor 647 was detected by flow cytometry. eGFP-LC3 assay MCF-7 eGFP-LC3 cells were seeded in 96-well plates and transfected the following day with indicated siRNA or miRNAs (50 nM). Three days after transfection, the cells were fixed in 4% formaldehyde and nuclei were stained with Hoechst (33342, lifetech). Bafilomycin A1 (Sigma-Aldrich) treatment was done 2 h before fixation (100 nM). Image acquisition was done using an Amersham InCell1000 High throughput microscope equipped with a × 40 Nikon objective. Fifteen pictures were taken from randomly placed positions within each well (counting ~1,000 cells per well) and analysed using the InCell1000 workstation 3.5 software package. Nuclei were segmented based on the Hoechst signal and cells were segmented from the GFP channel. Cells with more than five eGFP-LC3 puncta were considered GFP-LC3 puncta-positive cells. qRT–PCR analysis Total RNA from transfected cells was isolated using Trizol reagent (Invitrogen). qRT–PCR was performed using the TaqMan reverse transcription kit (Applied Biosystems) and Fast SYBR Green PCR Master Mix (Applied Biosystems). Primer sequences are shown in Supplementary Table 2 . Housekeeping genes used for normalization were Ubiquitin, RPO and 36B4. Human tissue RNA samples were purchased from Labinova AB, Sweden. miRNA qRT–PCR analysis was performed with TaqMan miRNA assays (Applied Biosystems). Small RNA housekeeping controls were miR-191, RNU44 and RNU6B. Affymetrix microarray processing MCF-7 cells were seeded in 6-cm plates and independent triplicate transfections were performed the following day with 50 nM miR-95 or scramble control. Total RNA was harvested 24 h after transfection using Trizol reagent and analysed by Affymetrix microarray analysis (HG-U133 Plus 2.0 Human). The microarray data have been submitted to the NCBI GEO database and assigned the identifier GSE58142. Background correction, between-array normalization and filtering steps were performed as previously described [21] . Differentially expressed genes were identified by a moderated t -test with FDR≤0.1 (1,336 transcripts and annotation as listed in Supplementary Table 1 ). We defined three data sets: downregulated set (1,087 transcripts) with FDR≤0.1 and log 2 FC<0, upregulated set (249 transcripts) with FDR≤0.1 and log 2 FC>0 and no change set containing randomly sampled 1,000 transcripts from the gene set with FDR>0.9. Luciferase reporter assays HEK cells were transfected in 96-well plates and luciferase activity was assessed 24–48 h after transfection by the Dual-Glo luciferase assay according to the manufacturer’s protocol (Promega). RLuc-based autophagic flux assay MCF-7 RLuc-LC3 WT and MCF-7 RLuc-LC3 G120A cells were reverse transfected with 50 nM siRNA or miRNA in RPMI without phenol red. Forty hours post transfection, 50 nM of Enduren substrate (Promega) was added and RLuc activity was measured at indicated time points. Antibodies and western blot analysis MCF-7, HEK or MSD cell lines were lysed in radioimmune precipitation buffer (150 mM NaCl, 1% Nonidet P-40, 0.5% sodium deoxycholate, 0.1% SDS, 50 mM Tris-HCl, pH 8, 2 mM EDTA) containing 1 mM dithiothreitol, 1 mM Pefabloc (Roche Applied Science), 1 × Complete Mini Protease Inhibitor Cocktail (Roche Applied Science), 1 × Phosphatase Inhibitor Cocktail (Roche Applied Science). Bafilomycin A1 treatment was 100 nM for 6 h before lysis. Protein (20–35 μg per lane) per lane was separated on a 4–12% NuPAGE Bis–Tris gel or at 16% (Invitrogen) Tris-Glycine gel and transferred to a nitrocellulose membrane or polyvinylidene difluoride membrane. The primary antibodies used were p62 (1:5,000, PM045, MBL), LC3 (1:200, M152-3, MBL), Ubiquitin (1:1,000, sc-8017, Santa Cruz), PARP (1:1,000, 9542, Cell Signaling), PSEN1 (1:250, MAB1563, Milipore), ATG2B (1:500, HPA019665, Sigma), Vinculin (1:100,000, V9131, Sigma) and GAPDH (1:20,000, sc-25778, Santa Cruz). The SUMF1 antibody (1:2,500) was kindly donated by Professor Thomas Dierks. The ARSB antibody (1:1000) was kindly provided by Dr Alberto Auricchio. Uncropped scans of selected original western blots are shown in Supplementary Fig. 6 . miRNAs/siRNAs/miRNA inhibitors and plasmids miRNAs and siRNA were miR-95 duplex (4427975, Life Technologies), Scramble (SIC001 mission siRNA Universal Negative Control #1, Sigma-Aldrich), siSUMF1 (smart pool L-019387-01-0005, Dharmacon). The control and miR-95 inhibitor plasmids were MZIP000-PA-1 and MZIP95-PA-1 (System Biosciences). pGL3‐SUMF1 was cloned by the PCR amplification of a 450-bp 3′UTR fragment from human genomic DNA and inserted into the pGL3 control vector (Invitrogen). Primers used for PCR amplification are as follows (restriction sites underlined): forward 5′- ggg- agatct- atgaagggatggacagcatg -3′ and reverse 5′- ggg- ctcgag -tagcgcacatttcacgttcg -3′. The quickchange site‐directed mutagenesis kit (Stratagene) was used for introducing three point mutations into the miR‐95-binding site, creating pGL3-SUMF1 MUT. The mutagenesis primer was 5′- gctgaagttcaggccttcaacacataggaatg -3′. The renilla luciferase vector pRLTK (Promega) was used for normalization. Plasmids PCDL-ARSA, PCDL-ARSC and pcDNA3-ARSB were previously described [12] , [32] . GAG assay Sulfated GAG content was measured using the Blyscan sulfated GAG assay kit according to the manufacturers protocol (Biocolor). In brief, this is a biochemical assay in which the 1,9-dimethylmethylene blue dye specifically labels sulfated GAGs. Samples were digested in a 0.2 M sodium phosphate buffer containing 8 mg ml −1 sodium acetate, 4 mg ml −1 EDTA, 0.8 mg ml −1 cysteine HCL and 0.1 mg ml −1 Papain (sigma) for 3 h at 65 °C with occasional mixing. The suspension was centrifuged at 10,000 g for 10 min and the supernatant was mixed with Blyscan dye reagent and shaken for 30 min at RT. Sulfated GAG-dye complexes were precipitated and collected by centrifugation and dissolved in Blyscan dissociation reagent. Absorbance was measured at 600 nm. Sulfatase enzymatic assays Specimens were disrupted by three freeze–thaw cycles. Protein concentration was measured in total homogenates. For all enzyme activity assays, 30 μg of protein was incubated at 37 °C for 3 h under the specific assay conditions. For the ARSA assay, homogenates were incubated with 0.05 M p -nitrocatechol sulfate in 0.25 M acetate buffer (pH 5) containing 0.85 M NaCl and 0.25 mM Na pyrophosphate in an incubation volume of 0.3 ml. The reaction was stopped with 0.7 ml 0.64 N NaOH, and the absorbance was read at 515 nm on a Perkin-Elmer spectrophotometer. For ARSB and ARSC enzymatic activity, 4-methylumbelliferyl (4-MU) sulfate was used as the substrate. ARSB and ARSC activity was determined by incubating cell homogenates with 6.25 mM 4-MU sulfate in 0.375 mM AgNO3, 0.1 M NaOAc buffer (pH 5) in 80 μl of incubation mixture. The reaction was stopped with 2 ml glycine-carbonate buffer (pH 10.7) and fluorescence was read at 365 nm (excitation) and 450 nm (emission) on a Turner fluorometer. Cathepsin B/L activity Cells were lysed 3 days after transfection in SCA lysis buffer (20 mM Hepes, 10 mM KCL, 1.5 mM EDTA, 1 mM EGTA and 250 mM sucrose) supplemented with 1 mM pefablock. For zFRase activity measurement, the lysate was mixed 1:1 with × 2 cathepsin reaction buffer (50 mM Na-acetate, 8 mM EDTA, 8 mM DTT, pH 5.0) supplemented with 1 mM pefablock and 20 μM cysteine cathepsin B and L substrate zFR-AFC (Enzyme Systems Products). V max of the liberation of the AFC fluorochrome from the substrate was measured with FLUOstar Optima (BMG LABTECH). The zFRase activity was normalized to the total protein concentration of the same sample. Transmission electron microscopy MCF-7 eGFP-LC3 cells were transfected as indicated for 72 h and treated with 200 nM rapamycin for the last 2 h before fixation in 2% v/v glutaraldehyde in 0.05 M sodium phosphate buffer (pH 7.2) for 24 h. Samples were rinsed three times in 0.15 M sodium cacodylate buffer (pH 7.2) and subsequently post-fixed in 1% w/v OsO 4 in 0.12 M sodium cacodylate buffer (pH 7.2) for 2 h. The specimens were dehydrated in a graded series of ethanol, transferred to propylene oxide and embedded in Epon according to standard procedures. Sections, B80-nm thick, were cut with a Reichert-Jung Ultracut E microtome and collected on copper grids with Formvar supporting membranes. Sections were stained with uranyl acetate and lead citrate. Imaging was done on a Phillips CM 100 BioTWIN transmission electron microscope. PTGui Pro digital imaging software was used for multiple image alignment of 24,500 × images to obtain high-resolution overview images of cellular cross-sections suitable for accurate identification and counting of autophagic vacuoles, mitochondria, early endosomes and multivesicular bodies. For each sample, 30–35 cellular cross-sections were counted and quantifications were calculated relative to cytoplasmic area. KEGG pathway analysis To identify the biological processes or pathways potentially regulated by miR-95, we applied the GeneCodis software analysis ( http://genecodis.cnb.csic.es ) on the list of 1,336 differentially expressed genes after miR-95 overexpression to identify enriched categories as defined by the KEGG pathways database. Categories with adjusted P values of 0.0001 or less are shown in Fig. 2b . For more information on this analysis, see refs 48 , 49 , 50 . Lentiviral transduction HEK cells were transfected with miRzip control or miR-95 inhibitor constructs together pAX8 (packaging) and pCMV-VSVG (envelope) plasmids and virus containing supernatants were harvested after 36 h. Supernatants were filtered through a 45-μm filter and supplemented with 8 μg ml −1 polybrene (Sigma). For adherent cells, virus supernatant was added to plated cells. For suspension cells (BA 1042 and BA 1043), the virus supernatant was added first to retronectin-coated plates followed by the addition of suspension cells. Cells were selected with 1–2 μg ml −1 puromycin (Invitrogen) 48 h after infection. Seed enrichment analysis We retrieved the annotated 3′UTR sequences of the transcripts on the microarrays from the UCSC table browser and included a unique 3′UTR for each transcript by choosing the one possessing the longest 3′UTR length. We searched seed sites of miR-95 against 3′UTR sequences of the up, down and no change sets. Four types of seed match were used as described [51] : 6mer (miRNA position 2 to 7), 7mer-m8 (miRNA position 2 to 8), 7mer-A1 (6mer plus nucleotide A at position 1) and 8mer (7mer-m8 plus nucleotide A at position 1). The significance of the proportional differences of the transcripts having seed sites in these three data sets was tested using two-sided Fisher’s exact test. Statistical analysis Unless otherwise indicated, all P values were calculated from a two-tailed Student’s t -test with equal variance. For all statistical analyses, P values are denoted as: *** P <0.0005, ** P <0.005 and * P <0.05. How to cite this article: Frankel, L. B. et al . A non-conserved miRNA regulates lysosomal function and impacts on a human lysosomal storage disorder. Nat. Commun. 5:5840 doi: 10.1038/ncomms6840 (2014).